Reprogramming of tRNA modifications controls the oxidative stress response by codon-biased translation of proteins Selective translation of survival proteins is an important facet of the cellular stress response. We recently demonstrated that this translational control involves a stress-specific reprogramming of modified ribonucleosides in tRNA. Here we report the discovery of a step-wise translational control mechanism responsible for survival following oxidative stress. In yeast exposed to hydrogen peroxide, there is a Trm4 methyltransferase-dependent increase in the proportion of tRNA Leu( C AA) containing m 5 C at the wobble position, which causes selective translation of mRNA from genes enriched in the TTG codon. Of these genes, oxidative stress increases protein expression from the TTG-enriched ribosomal protein gene RPL22A , but not its unenriched paralogue. Loss of either TRM4 or RPL22A confers hypersensitivity to oxidative stress. Proteomic analysis reveals that oxidative stress causes a significant translational bias towards proteins coded by TTG-enriched genes. These results point to stress-induced reprogramming of tRNA modifications and consequential reprogramming of ribosomes in translational control of cell survival. Decades of study have revealed more than 100 ribonucleoside structures incorporated as post-transcriptional modifications mainly in transfer RNA and ribosomal RNA, with 25–35 modifications present in any one organism [1] , [2] , [3] , [4] . In general, tRNA modifications enhance ribosome-binding affinity, reduce misreading and modulate frame shifting, all of which affect the rate and fidelity of translation [5] , [6] , [7] , [8] . Emerging evidence points to a critical role for tRNA and rRNA modifications in the various cellular responses to stimuli, such as tRNA stability [9] , [10] , transcription of stress response genes [11] , [12] , [13] and control of cell growth [14] . We recently used high-throughput screens and targeted analyses to show that the tRNA methyltransferase 9 (Trm9) modulates the toxicity of methylmethanesulfonate in Saccharomyces cerevisiae [12] , [15] . This is similar to the observed role of Trm9 in modulating the toxicity of ionizing radiation [16] and of Trm4 and other translation associated proteins in promoting viability after methylation damage [15] , [17] . Trm9 catalyses the methyl esterification of the uracil-based cm 5 U and cm 5 s 2 U to mcm 5 U and mcm 5 s 2 U, respectively, at the wobble positions of tRNA U CU -ARG and tRNA U UC -GLU, among others [18] . These wobble base modifications enhance binding of the anticodon with specific codons in mixed codon boxes [19] . Codon-specific reporter assays and genome-wide searches revealed that Trm9-catalysed tRNA modifications enhanced the translation of AGA- and GAA-rich transcripts that functionally mapped to processes associated with protein synthesis, metabolism and stress signalling [12] . These results lead to a model in which messenger RNA possessing specific codons will be more efficiently translated by tRNA, with anticodons containing the Trm9-modified ribonucleoside and that tRNA modifications can dynamically change in response to stress. To study the functional dynamics of this conserved system, we recently developed a bioanalytical platform to quantify the spectrum of ribonucleoside modifications and we used it to assess the role of RNA modifications in the stress response of S. cerevisiae [20] . This approach led to the discovery of signature changes in the spectrum of tRNA modifications in the cellular response to mechanistically different toxicants. Exposure of yeast to hydrogen peroxide (H 2 O 2 ), as a model oxidative stressor, led to increases in the levels of 2′- O -methylcytosine (Cm), 5-methylcytosine (m 5 C) and N 2 , N 2 -dimethylguanosine (m 2 2 G), whereas these ribonucleosides decreased or were unaffected by exposure to methylmethanesulfonate, arsenite and hypochlorite [20] . Loss of the methyltransferase enzymes catalysing the formation of the modified ribonucleosides led to cytotoxic hypersensitivity to H 2 O 2 exposure [20] . These results support a general model of dynamic control of tRNA modifications in cellular response pathways and expand the repertoire of mechanisms controlling translational responses in cells. In the present study, we have used a variety of bioanalytical and bioinformatic approaches to define a step-wise mechanistic link between tRNA modifications and the oxidative stress response. Following an oxidative stress, reprogramming of a specific tRNA wobble modification leads to selective translation of mRNA species enriched with the cognate codon. Among the codon-biased, selectively translated proteins is one member of a pair of ribosomal protein paralogues, and the loss of this paralogue causes sensitivity to oxidative stress. These results lead to a model in which stress-induced reprogramming of tRNA modifications and the associated reprogramming of ribosomes provides translational control of cell survival following an oxidative stress. H 2 O 2 increases m 5 C at the wobble position of tRNA Leu( C AA) In S. cerevisiae , m 5 C is synthesized by Trm4 methyltransferase (also called Ncl1) and we previously observed that the level of m 5 C in total tRNA increased following exposure to H 2 O 2 (ref. 20 ), with loss of Trm4 causing hypersensitivity to the cytotoxic effects of H 2 O 2 (ref. 20 ). To rule out second site mutations as the cause of this phenotype, we performed a complementation study using a TRM4 expression vector in the trm4 mutant strain and observed that re-expression of Trm4 conferred resistance to H 2 O 2 exposure ( Supplementary Fig. S1 and Supplementary Methods ). Although m 5 C is present in at least 34 species of tRNA [2] , tRNA Leu( C AA) is the only tRNA with m 5 C at the anticodon wobble position 34, as well as position 48 at the junction between the variable and TΨC loops [2] . To determine whether H 2 O 2 exposure altered the levels of m 5 C at one or both of these positions, tRNA Leu( C AA) was purified from H 2 O 2 -exposed and unexposed cells by sequential gel and affinity purification. The resulting purified tRNA Leu( C AA) was digested with RNase T1 to give a signature 4-mer oligoribonucleotide harbouring either C or m 5 C at position 48 ( C AAG) ( Fig. 1a ). In addition, total tRNA from H 2 O 2 -exposed and unexposed S. cerevisiae was digested with RNase U2 to produce another unique 5-mer oligoribonucleotide with C or m 5 C at position 34 of tRNA Leu( C AA) (UU C AA) ( Fig. 1a ). As shown in Fig. 1b , subsequent mass spectrometric analysis of these oligonucleotides revealed that H 2 O 2 exposure caused a 70% increase in m 5 C at the wobble position and a 20% decrease at position 48. 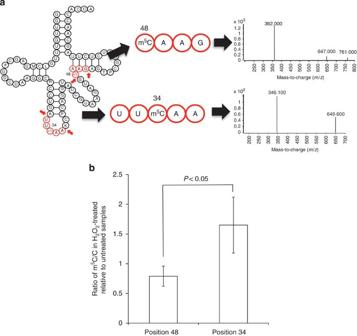Figure 1: H2O2exposure increases the level of m5C at the wobble position of tRNALeu(CAA). (a) tRNALeu(CAA)was digested with ribonucleases to generate oligoribonucleotides containing m5C or C at position 34 (CAAG) or position 48 (UUCAA), and the oligoribonucleotides were quantified by mass spectrometry. (b) The graph shows the ratio of m5C/C in tRNALeu(CAA)from H2O2-treated cells relative to untreated cells. The data represent mean±s.d. for three experiments. The data for position 34 are significantly different from those for position 48 by Student'st-test withP<0.05. Figure 1: H 2 O 2 exposure increases the level of m 5 C at the wobble position of tRNA Leu( C AA) . ( a ) tRNA Leu( C AA) was digested with ribonucleases to generate oligoribonucleotides containing m 5 C or C at position 34 ( C AAG) or position 48 (UU C AA), and the oligoribonucleotides were quantified by mass spectrometry. ( b ) The graph shows the ratio of m 5 C/C in tRNA Leu( C AA) from H 2 O 2 -treated cells relative to untreated cells. The data represent mean±s.d. for three experiments. The data for position 34 are significantly different from those for position 48 by Student's t -test with P <0.05. Full size image m 5 C controls the translation of UUG-enriched mRNA Next, we asked if the presence of m 5 C in tRNA Leu( C AA) enhanced the translation of UU G -containing mRNA, given the evidence that m 5 C at the wobble position of the leucine-inserting amber suppressor tRNA Leu( C UA) enhances translation [21] . To test this hypothesis, we used a dual Renilla and Firefly luciferase reporter construct [22] (illustrated in Fig. 2a ), in which the linker region connecting these two in-frame coding sequences was either four random or four TTG codons in a row (control and 4X-TTG, respectively). Expression of the Firefly luciferase portion of the reporter fusion protein is thus dependent upon the efficiency of translating the linker region [22] . The expression of both the Renilla and Firefly luciferase reporters was quantified under conditions of oxidative stress and loss of Trm4 activity ( Fig. 2b , Supplementary Fig. S2 ). As shown in Fig. 2b , loss of Trm4 caused a 9.6-fold reduction in 4X-TTG reporter expression relative to wild-type cells under basal conditions. Following H 2 O 2 treatment, there was an even larger 23.8-fold reduction in 4X-TTG reporter activity in trm4 Δ cells compared with wild-type cells, with 4X-TTG reporter expression in wild-type cells unaffected by H 2 O 2 exposure ( Fig. 2b ). Effects of this magnitude were not observed for the control reporter, which was devoid of TTG codons in the linker region ( Supplementary Fig. S2 ). The trm4 Δ cells containing the control reporter had an H 2 O 2 -induced twofold decrease in Firefly luciferase expression, relative to untreated cells, suggesting contributions by Trm4 to some aspect of general translation during oxidative stress. Taken together, these results are consistent with the idea that translation of TTG-rich sequences is facilitated by Trm4-catalysed tRNA modifications and that m 5 C modifications have an important role in the translational response to H 2 O 2 exposure. Coupled with the evidence for H 2 O 2 -induced increases in m 5 C at the wobble position of tRNA Leu( C AA) , the data support a model in which oxidative stress causes a Trm4-mediated increase in the incorporation of m 5 C in tRNA Leu( C AA) , with the methylated wobble base enhancing the translation of mRNA from genes enriched in TT G codon usage for leucine. 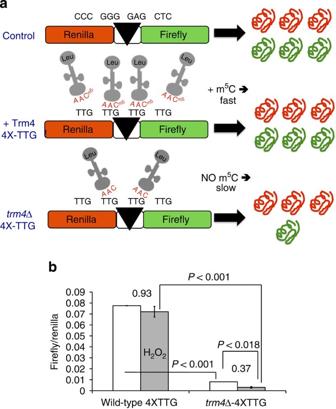Figure 2: H2O2and Trm4 methyltransferase control gene expression at the level of TTG codon usage. (a) Scheme illustrating the dual luciferase reporter system for assessing the effect of TTG codon usage on protein expression in wild-type andtrm4Δ mutant yeast cells transformed with either control or 4X-TTG reporter plasmids. (b) Control and 4X-TTG reporter activity was quantified in H2O2-exposed (grey bars) and unexposed (white bars) wild-type ortrm4Δ cells. The ratio of treated to untreated is indicated above each condition. Data represent mean±s.d. for three biological replicates. Figure 2: H 2 O 2 and Trm4 methyltransferase control gene expression at the level of TTG codon usage. ( a ) Scheme illustrating the dual luciferase reporter system for assessing the effect of TTG codon usage on protein expression in wild-type and trm4 Δ mutant yeast cells transformed with either control or 4X-TTG reporter plasmids. ( b ) Control and 4X-TTG reporter activity was quantified in H 2 O 2 -exposed (grey bars) and unexposed (white bars) wild-type or trm4 Δ cells. The ratio of treated to untreated is indicated above each condition. Data represent mean±s.d. for three biological replicates. Full size image Differential codon enrichment in genes for ribosomal protein paralogues This direct link between a tRNA wobble modification, codon usage and gene expression immediately raised the question of biases in the distribution of the TTG codon in genes that have a role in responding to oxidative stress. Using a recently developed S. cerevisiae codon distribution database [23] , we quantified TTG codon use across the yeast genome. An average of 29% of leucines are coded by TTG in the 5,782 genes analysed. However, in 38 genes, more then 90% of the leucines are coded by TTG. Intriguingly, among these 38 genes, 26 encoded ribosomal proteins and the others are loosely related to energy metabolism ( Table 1 ). These 26 ribosomal proteins represent a subset of the 138 such proteins encoded by the yeast genome. Of the 78 proteins that comprise a ribosome in S. cerevisiae , 59 occur in homologous pairs, or paralogues, that are believed to have arisen by an evolutionary genome duplication event [24] . Recent evidence supports a model in which individual paralogues have different functional roles in a variety of cell processes in yeast [25] , [26] , [27] , [28] , with studies by Komili et al . [29] revealing that a specific set of ribosomal protein homologues is necessary for the translation of ASH1 mRNA during bud tip formation. One striking feature of the genes encoding paralogous ribosomal proteins is a bias in frequency of TTG codon use, as shown in Supplementary Tables S1 and S2 . For example, 100% and 34% of the leucines in the paralogues Rpl22A and Rpl22B, respectively, are coded by TTG. Table 1 S. cerevisiae genes with ≥90% TTG codon usage for leucine. Full size table H 2 O 2 increases a TTG-enriched ribosomal protein paralogue The biased distribution of TTG codons in ribosomal protein paralogues raised another question: will H 2 O 2 -induced increases in m 5 C in tRNA Leu( C AA) lead to selective expression of TTG-enriched ribosomal protein paralogues? To test this hypothesis, we used a mass spectrometry-based proteomics approach to determine the relative quantities of several ribosomal protein paralogues in wild-type and trm4 Δ mutant yeasts exposed to H 2 O 2 . The study entailed isolation of polysomes from lysates of H 2 O 2 -treated and control yeast cells by differential ultracentrifugation, followed by trypsin digestion of the proteins and quantification of the tryptic peptides by liquid chromatography-coupled high-resolution mass spectrometry (LC-MS). Using this approach, we were able to consistently identify 39 ribosomal proteins in each of three biological replicates ( Supplementary Table S3 ), including seven pairs of distinguishable paralogues (Rpl6a/b, Rpl7a/b, Rpl16a/b, Rpl22a/b, Rpl33a/b, Rpl36a/b and Rps7a/b) ( Supplementary Tables S3 and S4 ). Although the amino-acid sequences of each set of paralogous proteins are nearly identical, they contain at least one signature tryptic peptide that could be used to identify and quantify each of 14 ribosomal paralogues in the mixture ( Supplementary Table S4 ). A protein BLAST search in the NCBI database using these peptide sequences confirmed that the peptides were unique to the specific S. cerevisiae ribosomal proteins (data not shown). Further, the sequence identity of these unique peptides was confirmed by the analysis of the b- and y-ion series in collision-induced dissociation (CID) spectra ( Supplementary Fig. S3 ). This approach was applied to determine the relative quantities of ribosomal homologues Rpl22a and Rpl22b, in which 100% and 34% of the leucines were coded by TTG, respectively. In the absence of absolute quantification of individual proteins, changes in the protein levels are expressed as changes in the ratio of the signals for the signature peptides from the protein pairs (for example, Rpl22a/Rpl22b). The LC-MS signal ratios for the 14 ribosomal paralogues are shown in Supplementary Tables S5 and S6 . A comparison of wild-type and trm4 Δ mutants revealed that loss of TRM4 caused a significant decrease in the ratio of Rpl22a to Rpl22b and of Rpl16b to Rpl16a ( Fig. 3 ), the two sets of paralogues with the largest differences in TTG codon use ( Supplementary Table S4 ). When wild-type and trm4 cells were exposed to H 2 O 2 , the ratio of Rpl22a to Rpl22b increased significantly in the wild-type cells but not in the trm4 mutants ( Fig. 4 ). To determine whether these changes are indeed occurring at the level of translation, we quantified mRNA for both Rpl22a and Rpl22b by real-time quantitative PCR and we observed that the transcript levels remained unchanged following loss of TRM4 or exposure to H 2 O 2 ( Supplementary Table S7 ). 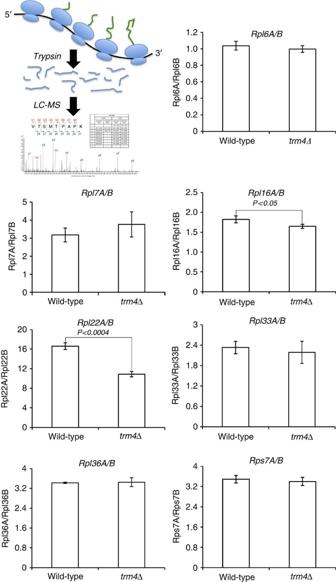Figure 3: Loss of Trm4 methyltransferase decreases the proportion of ribosomes containing TTG codon-enriched ribosomal protein paralogues. Ribosomal proteins in wild-type andtrm4Δ mutantS. cerevisiaewere quantified by LC-MS/MS (schematic inset) and the relative quantities of ribosomal protein paralogues presented as the ratio of the signal intensity for the paralogue with high TTG usage to that of the low-usage paralogue. Data represent mean±s.d. for three biological replicates.Pvalues denote statistically significant differences by Student'st-test. Figure 3: Loss of Trm4 methyltransferase decreases the proportion of ribosomes containing TTG codon-enriched ribosomal protein paralogues. Ribosomal proteins in wild-type and trm4 Δ mutant S. cerevisiae were quantified by LC-MS/MS (schematic inset) and the relative quantities of ribosomal protein paralogues presented as the ratio of the signal intensity for the paralogue with high TTG usage to that of the low-usage paralogue. Data represent mean±s.d. for three biological replicates. P values denote statistically significant differences by Student's t -test. 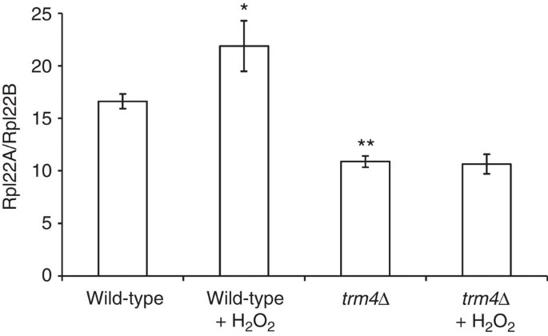Figure 4: H2O2exposure increases the proportion of ribosomes containing ribosomal protein paralogue Rpl22a in wild-typeS. cerevisiaebut not intrm4Δ mutants. Cells were exposed to 2 mM H2O2for 1 h and the quantities of ribosomal proteins were determined by LC-MS/MS analysis. Data are expressed as the ratio of the TTG-enriched paralogue Rpl22a to unenriched Rpl22b. Data represent mean±s.d. of three biological replicates. Asterisks denote statistically significant differences between H2O2-treated and untreated cells as judged by Student'st-test withP<0.05. Full size image Figure 4: H 2 O 2 exposure increases the proportion of ribosomes containing ribosomal protein paralogue Rpl22a in wild-type S. cerevisiae but not in trm4 Δ mutants. Cells were exposed to 2 mM H 2 O 2 for 1 h and the quantities of ribosomal proteins were determined by LC-MS/MS analysis. Data are expressed as the ratio of the TTG-enriched paralogue Rpl22a to unenriched Rpl22b. Data represent mean±s.d. of three biological replicates. Asterisks denote statistically significant differences between H 2 O 2 -treated and untreated cells as judged by Student's t -test with P <0.05. Full size image H 2 O 2 enhances translation of proteins with TTG-enriched genes Having performed a targeted analysis of ribosomal proteins that revealed evidence of selective translation of TTG-enriched proteins, we next undertook a more general proteomic analysis of H 2 O 2 -induced differences in the ~200 most abundant proteins in yeast ( Supplementary Data 1 ), using a SILAC-based approach to quantify changes in the abundance of proteins in H 2 O 2 -induced cells [30] . As shown in Fig. 5 , proteins with high TTG usage are more likely to be downregulated ( Fig. 5a , P =0.048 by Student's t -test) as a consequence of loss of Trm4 activity, whereas these proteins are significantly upregulated in wild-type cells exposed to H 2 O 2 ( Fig. 5b , P =6.41×10 −7 ). However, oxidative stress did not affect the expression of proteins from TTG-enriched genes in trm4 Δ cells ( Fig. 5c , P =0.554), which is consistent with a role for m 5 C in the selective translation of UUG-enriched mRNA species. 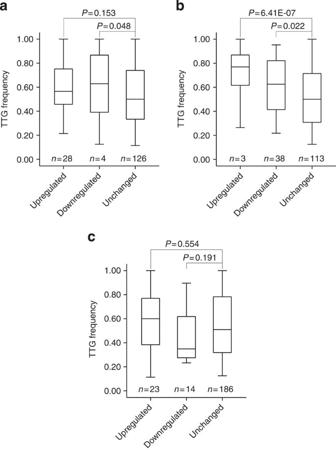Figure 5: SILAC-based proteomic analysis reveals that H2O2enhances the translation of TTG-enriched proteins. Protein extracts from control and H2O2-treated wild-type andtrm4mutant yeast were mixed 1:1 with proteins from U-[13C,15N]-lysine-labeledlys1Δ yeast cells as an internal standard30. Protein mixtures were then subjected to trypsin digestion and proteomic analysis by LC-QTOF analysis. The quantities of the 261 most abundant proteins appearing in each of four biological replicates were analysed by Student'st-test (P<0.05) for increased (upregulation), decreased (downregulation) or unchanged levels in (a)trm4Δ mutant versus wild-type cells, (b) H2O2-treated versus untreated wild-type cells, and (c) H2O2-treated versus untreatedtrm4Δ mutant cells. Within these three groups of proteins, the frequency of using TTG to code for leucine was calculated. The resulting frequency data are presented as a box-and-whiskers plot with the bar representing the median value, the box encompassing the range of data between the first and third quartile, and the error bars embracing data within 1.5-times interquartile range. Differences between upregulated, downregulated and unchanged categories were subjected to Student'st-test with the indicatedPvalues. Figure 5: SILAC-based proteomic analysis reveals that H 2 O 2 enhances the translation of TTG-enriched proteins. Protein extracts from control and H 2 O 2 -treated wild-type and trm4 mutant yeast were mixed 1:1 with proteins from U-[ 13 C, 15 N]-lysine-labeled lys1 Δ yeast cells as an internal standard [30] . Protein mixtures were then subjected to trypsin digestion and proteomic analysis by LC-QTOF analysis. The quantities of the 261 most abundant proteins appearing in each of four biological replicates were analysed by Student's t -test ( P <0.05) for increased (upregulation), decreased (downregulation) or unchanged levels in ( a ) trm4 Δ mutant versus wild-type cells, ( b ) H 2 O 2 -treated versus untreated wild-type cells, and ( c ) H 2 O 2 -treated versus untreated trm4 Δ mutant cells. Within these three groups of proteins, the frequency of using TTG to code for leucine was calculated. The resulting frequency data are presented as a box-and-whiskers plot with the bar representing the median value, the box encompassing the range of data between the first and third quartile, and the error bars embracing data within 1.5-times interquartile range. Differences between upregulated, downregulated and unchanged categories were subjected to Student's t -test with the indicated P values. Full size image Analysis of the functional categories of proteins affected by H 2 O 2 exposure ( Supplementary Fig. S4 ) reveals that proteins related to translation are significantly upregulated by oxidative stress, which is consistent with the analysis of ribosomal protein expression in Fig. 4 , although Rpl22A and Rpl22B could not be differentiated likely as a result of the minimal sequence difference between the two proteins. One interesting complication apparent in Fig. 5b is that proteins from genes with intermediate TTG frequencies (that is, frequencies between the unchanged and upregulated fractions) are significantly downregulated in both H 2 O 2 -exposed wild-type cells ( P =0.022) and trm4 Δ mutants ( P =0.048). This illustrates the limitations of our model for selective expression of TTG-enriched genes following oxidative stress and suggests that other layers of translational control are operant in the response to H 2 O 2 exposure. Rpl22A is required for the oxidative stress response in yeast To further refine the mechanistic link between H 2 O 2 exposure, m 5 C modification of tRNA and Rpl22A expression as a survival response, we assessed the H 2 O 2 sensitivity of yeast strains lacking individual Rpl16A/B and Rpl22A/B paralogues. As shown in Fig. 6 , only the loss of RPL22A conferred sensitivity to H 2 O 2 , whereas the loss of RPL16A , RPL16B and RPL22B did not affect H 2 O 2 -induced cytotoxicity. The magnitude of the increased cytotoxicity caused by loss of Rpl22A (20 to 10% survival) is similar to the change in cytotoxicity that we observed previously for loss of Trm4 (ref. 20 ). This suggests that Rpl22A contributes significantly to the oxidative stress survival response in yeast. The lack of effect of Rpl16b loss on H 2 O 2 toxicity, in spite of the Trm4-dependence of this TTG-enriched paralogue ( Fig. 3 ), suggests that it shares functional equivalence with Rpl16a in ribosomes. 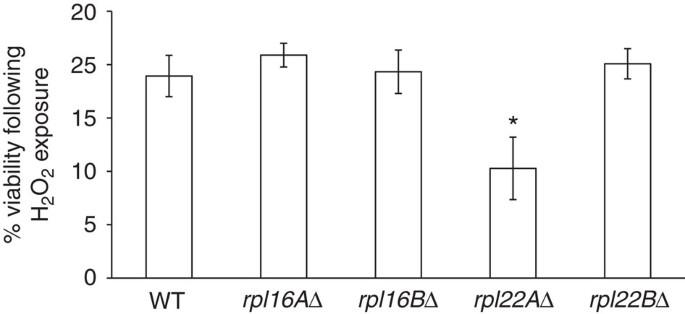Figure 6: Ribosomal protein paralogue Rpl22a confers resistance to H2O2exposure inS. cerevisiae. Wild-type (WT)S. cerevisiaeand strains lackingRPL16A,RPL16B, RPL22AorRPL22Bwere exposed to 5 mM H2O2and survival was assayed as described in Methods. Data represent mean±s.d. of three biological replicates. The asterisk denotes a statistically significant difference compared with all other values in the figure, as judged by Student'st-test withP<0.05. Figure 6: Ribosomal protein paralogue Rpl22a confers resistance to H 2 O 2 exposure in S. cerevisiae . Wild-type (WT) S. cerevisiae and strains lacking RPL16A , RPL16B, RPL22A or RPL22B were exposed to 5 mM H 2 O 2 and survival was assayed as described in Methods. Data represent mean±s.d. of three biological replicates. The asterisk denotes a statistically significant difference compared with all other values in the figure, as judged by Student's t -test with P <0.05. Full size image Using a combination of bioanalytical and bioinformatic tools, we have defined a step-wise translational control mechanism responsible for cell survival following oxidative stress, a model for which is shown in Fig. 7 . Although some of the individual steps in this model could be explained by other phenomena, such as tRNA or protein stability, there are few, if any, alternative mechanisms that could explain the sum of the observed behaviours. The first step in this model involves H 2 O 2 -induced increases in the level of m 5 C at the wobble position of tRNA Leu( C AA) ( Fig. 7a ) with a concomitant decrease in m 5 C at the neighbouring position 48 in the same tRNA. The observation of a 70% increase in the proportion of tRNA Leu( C AA) molecules containing a wobble m 5 C is consistent with a simple increase in TRM4 activity acting on a fixed concentration of total tRNA Leu( C AA) . Alternatively, the proportion of m 5 C-containing tRNA Leu( C AA) could remain constant, with an increase in transcription leading to an increase in the total number of copies of tRNA Leu( C AA) , or both transcription and TRM4 activity could increase to raise the concentration of tRNA Leu( C AA) with m 5 C. Finally, given the precedent for stress-induced degradation of tRNA [9] , [10] , oxidative stress could lead to selective degradation of unmethylated tRNA Leu( C AA) . By any mechanism, the data show that oxidative stress increases the proportion of tRNA Leu( C AA) containing m 5 C at the wobble position, with an absolute requirement for Trm4 activity for the existence of m 5 C [20] . 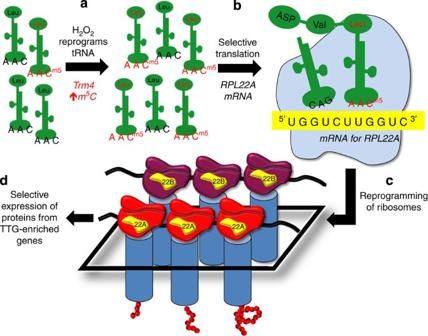Figure 7: Proposed mechanism by which increase in m5C level regulates translation of ribosomal protein paralogues and confers resistance to H2O2. Exposure to H2O2leads to an elevation in the level of m5C at the wobble position of the leucine tRNA for translating the codon UUG on mRNA (a), which enhances the translation of the UUG-enrichedRPL22AmRNA relative to its paralogueRPL22B(b) and leads to changes in ribosome composition (c). This reprogramming of tRNA and ribosomes ultimately causes selective translation of proteins from genes enriched with the codon TTG (d). Figure 7: Proposed mechanism by which increase in m 5 C level regulates translation of ribosomal protein paralogues and confers resistance to H 2 O 2 . Exposure to H 2 O 2 leads to an elevation in the level of m 5 C at the wobble position of the leucine tRNA for translating the codon UUG on mRNA ( a ), which enhances the translation of the UUG-enriched RPL22A mRNA relative to its paralogue RPL22B ( b ) and leads to changes in ribosome composition ( c ). This reprogramming of tRNA and ribosomes ultimately causes selective translation of proteins from genes enriched with the codon TTG ( d ). Full size image The second step in the model posits that the increase in m 5 C in tRNA Leu( C AA) enhances the efficiency of translation of mRNAs enriched in the UUG codon recognized by this tRNA ( Fig. 7b ). This is supported by the reporter assay results shown in Fig. 2 , with loss of Trm4 activity having no or little effect on reporter expression when TTG usage is low but causing a sharp decrease in expression when TTG usage is high. This is consistent with the observation that loss of Trm4, and thus m 5 C, decreases the expression of TTG-enriched proteins but not unenriched proteins ( Figs 3 and 5 ). The observation using the unmodified reporter ( Supplementary Fig. S2 ) that H 2 O 2 exposure of wild-type cells did not affect reporter expression levels, yet it decreased reporter expression in the trm4 Δ mutant, points to contributions by factors other than modification-specific codon usage in the control of translation during the oxidative stress response. In addition to the proteome changes shown in Fig. 5 , the observed changes in expression of ribosomal proteins Rpl22A and Rpl16B ( Figs 3 and 4 ) are consistent with the idea that oxidative stress enhances the translation of UUG-biased mRNAs. The pair of ribosomal gene parologues with the widest difference in the use of TTG for coding leucine, RPL22A at 100% and RPL22B at 38%, showed the largest changes in protein expression following H 2 O 2 exposure, with expression of the high TTG usage RPL22A increasing with oxidative stress and decreasing with loss of TRM4 ( Fig. 4 ). The latter result points to the translational control of Rpl22A by Trm4, with the absolute requirement of oxidation-induced increases in m 5 C for the enhanced expression of Rpl22A. Although we cannot rule out differential protein stability as a determinant of the proportions of the ribosomal protein paralogues, differences in leucine content do not account for the differential stability of Rpl22A and Rpl22B. The paralogues differ minimally in leucine content and the changes in paralogue levels caused by loss of TRM4 do not correlate with this amino acid. Although Rpl22A and Rpl22B have 7 and 8 leucines, respectively, and the relative amount of Rpl22A decreases with loss of TRM4, Rpl16A and Rpl16B have 17 and 18 leucines, respectively, yet the relative quantity of RPL16A decreases with loss of TRM4. Further, the data presented here do not provide insights into the function of ribosomes with TTG-enriched ribosomal proteins, such as their potential role in selective translation of mRNAs enriched with TTG or other codons, or their possible role in the early and late stages of the oxidative stress response. A detailed analysis of ribosome-bound mRNAs or nascent peptides in the early and late stages of the oxidative stress response would shed light on these issues. When considered with the other results, our observations suggest that the H 2 O 2 -induced increase in the level of the Rpl22a ribosomal protein is caused, at least in part, by Trm4-mediated changes in m 5 C levels in tRNA with subsequent control of translation of mRNA arising from TTG-enriched genes. The mechanistic connection between Trm4 and Rpl22A is further established by the observation that loss of either protein makes corresponding trm4 Δ [20] or rpl22a Δ ( Fig. 6 ) cells sensitive to H 2 O 2 . There are parallels for the H 2 O 2 -sensitive phenotype of rpl22a Δ in the recently defined roles of other ribosomal proteins in the oxidative stress response in higher eukaryotes. One example also serves as an illustration of the ribosome filter hypothesis concerning selective translation of mRNA [31] : human ribosomal protein Rpl26 regulates translation of p53, a major node in oxidative stress response [32] , by interacting with the 5′-untranslated region of p53 mRNA [33] . Similarly, the highly conserved Rpl22 (ref. 34 ) is involved in the activation of internal ribosomal entry site-mediated translation in response to several types of stress [35] , [36] and it participates in murine T-cell development by regulating translation of p53 (ref. 37 ). Interestingly, ribosomal proteins may have roles in stress response other than ribosome structure, as suggested by recent observations of Rpl22 involvement in non-ribosomal ribonucleoprotein complexes such as the telomerase holoenzyme [36] , [38] , [39] , [40] . This series of observations leads to a model ( Fig. 7 ) in which oxidative stress causes an early increase in Trm4-mediated m 5 C levels in tRNA Leu( C AA) , which leads to selective translation of UUG-enriched mRNAs, including ribosomal protein paralogue Rpl22a and other proteins derived from many TTG-enriched genes. Clearly, this model does not address the complexity of translational control mechanisms, as suggested by the proteomic analysis shown in Fig. 5 , in which mRNA from genes with varying enrichment of TTG codons are not necessarily subject to enhanced translational efficiency. This complexity is further illustrated by the possibility of reprogramming of other modifications, such as H 2 O 2 -induced increases in Cm and m 2 2 G [20] , in other tRNA species, with subsequent selective expression of mRNAs enriched with other codons, as well as the potential for reprogramming of ribonucleoside modifications in rRNA species. Nonetheless, the present observations add to the growing recognition of a role for functional diversity in ribosome composition [41] and a role for ribosomes in selective translation of proteins [31] . This reconfiguration of the translation machinery is similar to the proposed generation of 'immunoribosomes' as a subset of T-cell ribosomes responsible for translating peptides involved in antigen presentation [42] . The abundance of ribosomal protein paralogues, the variety of RNA modifications in tRNA and rRNA, and the established biases in codon distributions in genes suggest a mechanism capable of fine tuning the translational response to virtually any cell stimulus. Codon reporter assay The effect of TTG codon frequency on protein expression in wild-type and trm4 Δ yeast cells was assessed using a dual luciferase reporter system [22] in which Renilla luciferase is connected in-frame to Firefly luciferase by a 12-bp sequence (control: 5′-CCCGGGGAGCTC-3′ or 4X-TTG: 5′-TTGTTGTTGTTG-3′), all under the control of an ADH1 promoter and CYC1 terminator [22] . Following transformation with either control or 4X-TTG plasmid, cells were grown to ~5×10 6 cells per ml and then treated with 2 mM H 2 O 2 or H 2 O for 60 min. Cell pellets were lysed by bead-beating in lysis buffer and lysates clarified by centrifugation. Luminescence reactions were initiated with Promega DLR (50 μl; Promega; Madison, WI) added to clarified lysates (5 μl) and measured using a Victor Plate Reader (PerkinElmer; Waltham, MA). RNase digestion of tRNA Purified tRNA Leu( C AA) (~2.5 μg) was digested with RNase T1 (1 U; Ambion, Austin, TX) in 10 mM Tris buffer (pH 7.4, 37 °C, 1 h). RNase U2 (Thermo Scientific, Waltham, MA) digestion (4 U) was carried out using total tRNA (0.5 mg, 37 °C, 4 h). Oligoribonucleotides were dephosphorylated with alkaline phosphatase (10 U). Quantifying m 5 C in tRNA Leu( C AA) RNase T1 and U2 digestion maps of tRNA were obtained using the Mongo Oligo Mass Calculator (v2.06; http://library.med.utah.edu/masspec/mongo.htm ). Digested tRNA oligos were resolved by HPLC (C18 Hypersil GOLD aQ, 150×2.1 mm, 3 μm particle; Thermo Scientific) coupled to a triple quadrupole mass spectrometer (MS; 6410; Agilent Technologies, Santa Clara, CA) with an electrospray ionization source operated in negative ion mode. HPLC was performed with a gradient of acetonitrile in 8 mM ammonium acetate (0.2 ml min −1 , 45 °C): 0–2 min, 1%; 2–30 min, 1–15%; 30–31 min, 15–100%; 31–41 min, 100%. MS parameters: drying gas, 325 °C and 8 l min −1 ; nebulizer, 30 p.s.i. ; capillary voltage, 3,800 V; dwell time, 200 ms. The first and third MS quadrupoles were set to unit resolution and the oligos containing m 5 C were identified by comparison with standards and CID fragmentation patterns generated in a quadrupole time-of-flight MS. A selected ion chromatogram for a particular charge state of each oligo (unexposed and exposed to H 2 O 2 ) was obtained, and the summation of the mass spectra over a particular peak was used for relative quantification of changes in m 5 C levels at positions 34 and 48 of tRNA Leu( C AA) . Ribosome isolation Cells (10 10 ) were resuspended in lysis buffer (10 ml) with 50 mM Tris-acetate, 50 mM ammonium chloride, 12 mM MgCl 2 and 1 mM dithiothreitol (pH 7) and lysed mechanically by bead-beating. Cell lysate was centrifuged (10,000 g , 10 min), the supernatant collected, and centrifugation repeated twice to remove all particulates. The debris-free supernatant was layered over 2.5 ml of 1 M sucrose, 20 mM HEPES, 500 mM KCl, 2.5 mM magnesium acetate and 2 mM dithiothreitol at pH 7.4 and centrifuged for 110 min at 370,000 g ( r max ). Supernatant was removed and the pelleted ribosomes were resuspended in 1.5 ml of a digestion buffer with 100 mM ammonium acetate, pH 8.5. The samples were concentrated by spin dialysis on YM-10 filters. The concentrate was re-diluted with the digestion buffer and subject to spin dialysis five times to remove salts. Yield: ~300 μg of protein. Identification of ribosomal proteins As the sequences of ribosomal protein paralogues are similar, we identified a unique tryptic peptide to quantify each paralogue. Following reduction with dithiothreitol (1 mM, 2 h, 37 °C) and alkylation with iodoacetamide (5.5 mM, 30 min, ambient temparture), purified ribosomal proteins (50 μg) were digested with proteomics-grade trypsin (1 μg) in 200 μl of ammonium acetate solution (100 mM, pH 8.5, 37 °C, 12 h). Samples were lyophilized and resuspended in 100 μl of 0.1% formic acid. Peptides in a portion of the tryptic digest (2.5 μg, 5 μl) were analysed by LC-MS on an Agilent 1200 capillary HPLC coupled to an Agilent 6520 QTOF MS (Agilent Technologies). Peptides were resolved on an Agilent ZORBAX 300SB-C18 column (100×0.3 mm, 3 μm particle) eluted with a gradient of acetonitrile in 0.1% formic acid (20 μl min −1 , 45 °C): 0–25 min, 1–30%; 25–30 min, 30–60%; 30–31 min, 60–95%; 31–36 min, 95%. The MS was operated in positive ion mode with electrospray parameters as follows: fragmentor voltage, 110 V; drying gas, 300 °C and 5 l min −1 ; nebulizer, 20 p.s.i. ; capillary voltage, 3,500 V. Peptide ions were scanned over m/z =100–1,700 at an acquisition rate of 1.4 spectra s −1 . Data analysis was performed with Agilent Mass Hunter Software and compounds were detected using molecular feature extractor with 300 count minimum peak height and maximum charge state of 2. The molecular feature extractor compound lists were subjected to peptide mass fingerprint analysis with the Agilent Spectrum Mill proteomics software to identify proteins based on peptide accurate mass. A search was performed against the NCBInr protein sequence database for S. cerevisiae with no protein modifications and missed cleavage considered, and with a 20 p.p.m. mass tolerance and >25% protein coverage. Identified peptides were sequenced by LC-coupled quadrupole time-of-flight (QTOF) mass spectrometry using HPLC conditions described earlier and operating the QTOF in targeted tandem mass spectroscopy (MS/MS) mode with acquisition rates for both MS and MS/MS scans at 1.4 spectra s −1 and a constant collision energy of 15 V to selectively monitor ions of the peptides shown in Supplementary Table S4 ; other MS parameters were described earlier. Peptide CID spectra were acquired by targeted MS/MS analysis and the b- and y-ion assignments ( Supplementary Fig. S3 ) used to determine the amino-acid sequence. A search of the NCBInr protein sequence database confirmed that each peptide uniquely identified its corresponding ribosomal protein paralogue. Relative quantification of ribosomal protein paralogues With unique tryptic peptides for each paralogue ( Supplementary Table S4 ), the selected ion chromatogram of each peptide at charge state +2 was extracted from the total ion chromatogram, with the MS signal intensity determined by summation of the area under the mass spectrum ( Supplementary Tables S5 and S6 ). Signal intensities for the ribosomal protein paralogues were normalized by taking their ratio, with the high TTG paralogue in the numerator and low TTG in the demoninator ( Supplementary Tables S5 and S6 ). This ratio was then used to determine changes in the quantities of ribosomal protein paralogues in H 2 O 2 -exposed cells ( Figs 3 and 4 ). SILAC proteomics Lys1 Δ yeast cells were grown in yeast nitrogen base medium containing 30 mg l −1 of L -lysine-U-[ 13 C] 6 , [ 15 N] 2 (Isotec-SIGMA, Miamisburg, OH) for ≥10 generations, until they reached log-phase (OD 600 ~0.7) [43] . Wild-type and trm4 Δ yeast cells were grown in yeast nitrogen base medium containing 30 mg l −1 of L -lysine and were treated with 5 mM H 2 O 2 at log-phase [20] . Cells were collected by centrifugation (1,500 g , 10 min, 4 °C), and washed twice with ice-cold H 2 O. Cells were lysed by suspension in 2 M NaOH, 8% 2-mercaptoethanol (v/v). Following TCA precipitation, proteins were pelleted by centrifugation (15,000 g , 15 min, 4 °C) and the pellet was resuspended in 8 M urea, 75 mM NaCl, 50 mM Tris, pH 8.2, 50 mM NaF, 50 mM β-glycerophosphate, 1 mM sodium orthovanadate, 10 mM sodium pyrophosphate and 1 mM phenylmethylsulphonyl fluoride [44] . Protein concentration was determined by the Bradford assay [45] . Heavy SILAC-labeled lys1 Δ yeast proteins were used as a global internal standard [30] . Following addition of internal standard to all treated and untreated wild-type and trm4 Δ yeast protein samples (1:1), the protein mixture was reduced in 1 mM dithiothreitol (2.5 h, 37 °C), alkylated with iodoacetamide (5.5 mM, 40 min, ambient temperature, dark) and then digested with 50:1 (w/w) trypsin (14 h, 37 °C). Peptide mixtures were loaded onto a Vydac C18 trap column (150 μm×10 mm, 5 μM, 300 Å particle; Grace, Deerfield, IL) at 5 μl min −1 and eluted onto a Vydac C18 analytical column (75 μm×150 mm, 5 μm per 300 Å particle) at 200 nl min −1 with a 120 min gradient of 2–98% acetonitrile in 0.1% formic acid. Eluted peptides were analysed by MS analysis on a QSTAR-XL (Applied Biosystems, Foster City, CA). Acquired MS/MS spectra were parsed by Spectrum Mill and searched against Swiss-Prot database. CID spectra of tryptic peptides were searched against the database sequences within a mass window of 100 p.p.m. for precursor ion searches and 500 p.p.m. for fragment ions. Database search results were filtered based on Spectrum Mill scoring criteria, which include peptide score, a measure of confidence of identification, and scored peak intensity (SPI) that represents the percentage of assigned peaks in CID spectrum. Peptide search results with a score ≥6, SPI≥60% and no missed cleavages were used for protein quantification. SILAC peptide and protein quantification was performed with differential expression quantification and SILAC protein ratios were determined as the average of all peptide ratios assigned to the protein. Differential protein expression was determined by Student's t -test for four biological replicates. A summary of identified proteins and their expression levels are presented in Supplementary Data 1 . The proteomics data has been deposited in the PeptideAtlas database ( http://www.peptideatlas.org/ ) under the accession code PASS00059 . Gene ontology annotation Gene functional categorization and pathway analysis were performed with DAVID Bioinformatics Resources 2011 (ref. 46 ). The annotated proteins are clustered according to the biological process branch of the GO annotation. The statistical significance of over-representation or under-representation of proteins in each GO category was assessed using a hypergeometric distribution and the significance indicated by the P values for each GO category. Accession codes: The proteomics data have been deposited in the PeptideAtlas database ( www.peptideatlas.org ) under the accession code PASS00059 . How to cite this article: Chan, C.T.Y. et al . Reprogramming of tRNA modifications controls the oxidative stress response by codon-biased translation of proteins. Nat. Commun. 3:937 doi: 10.1038/ncomms1938 (2012).